Holographic optogenetic stimulation of patterned neuronal activity for vision restoration When natural photoreception is disrupted, as in outer-retinal degenerative diseases, artificial stimulation of surviving nerve cells offers a potential strategy for bypassing compromised neural circuits. Recently, light-sensitive proteins that photosensitize quiescent neurons have generated unprecedented opportunities for optogenetic neuronal control, inspiring early development of optical retinal prostheses. Selectively exciting large neural populations are essential for eliciting meaningful perceptions in the brain. Here we provide the first demonstration of holographic photo-stimulation strategies for bionic vision restoration. In blind retinas, we demonstrate reliable holographically patterned optogenetic stimulation of retinal ganglion cells with millisecond temporal precision and cellular resolution. Holographic excitation strategies could enable flexible control over distributed neuronal circuits, potentially paving the way towards high-acuity vision restoration devices and additional medical and scientific neuro-photonics applications. In principle, direct photo-stimulation offers the ability to control distributed neuronal circuits with cellular resolution. This could be highly desirable for neuro-photonic applications of optogenetic technology [1] , [2] including optogenetic retinal prostheses [3] , [4] , [5] , [6] , [7] , [8] , [9] , because sensory information is generally represented in distributed spatio-temporal patterns of activity carried across large populations of neurons, while neighbouring neurons in real circuits are often found to have widely divergent response properties. Although electrical retinal prostheses are already being used to aid blind human subjects, it appears that their ultimate performance/resolution may be limited by current spread, and the acuity of ~20/2,000 is common to both 60 electrode epiretinal and 1,500 electrode sub-retinal systems. A pattern photo-stimulation system for artificially controlling neural activity in a vision prosthesis or for general neuro-stimulation applications is not expected to have this limitation (due to minimal light scattering in the inner retinal layers) and will ideally allow cellular-resolution, rapid, massively parallel, light-efficient stimulation across macroscopic (millimeter-scale) coverage areas. To date, however, optical excitation of optogenetically targeted populations is often delivered non-specifically to the whole population using wide-field flashes with intense lamps [1] , [3] , [10] , LEDs (light-emitting diodes) and optical fibre coupled illumination [11] , [12] or in simple patterns using rapid random-access laser deflection [13] , [14] , digital micromirror arrays [8] , [9] , [15] , [16] , [17] , [18] and micro-LED arrays [6] , [19] . Diffractive wavefront shaping techniques including computer-generated holography (CGH) and generalized phase contrast are an emerging tool for dynamic patterned photo-excitation [20] , [21] , [22] , [23] that were shown to allow structured two-(2D) and three-dimensional (3D) excitation of dendritic arbors [20] , [24] and neurons [25] using neurotransmitter photolysis as well as two-photon optogenetic stimulation of several neurons in brain slices [26] . The principle advantage of CGH systems [22] , [23] is that they naturally combine the high intensity, efficiency and resolution that are characteristic of sequential laser deflection methods (such as acousto-optical deflectors) with the capacity for scan-less simultaneous parallel illumination of multiple locations of micro-display array projectors, but without their respective limitations. That is, unlike digital mirrors and other array microdisplays, CGH divides power among the ‘on’ stimulation pattern and avoids the massive inefficiency resulting from blocking the light to the large proportion of ‘off’ pixels (typically >>90%), and unlike laser deflectors, the patterns are projected simultaneously rather than sequentially, and are thus independent of (the relatively long) dwell times. Although CGH has multiple advantageous properties as a photo-stimulation tool, previous direct demonstrations of single-photon CGH were limited to neurotransmitter photolysis in brain slices [20] , [24] , [25] and were strongly limited in their speed, stimulation field (SF) area and number of simultaneously activated neurons. To fully realize the millisecond-timescale dynamical controllability of optogenetic probes, we developed a rapid CGH photo-stimulation system based on a fast-switching ferroelectric liquid-crystal spatial light modulator (SLM) [27] , which can practically switch patterns in kHz rates. Such rapid CGH systems could also use their high projection rates to effectively average-out holographic speckle noise without adding to the computational burden associated with these systems [28] . Here, we demonstrate and study the performance and characteristics of rapid CGH as a tool for large-scale, cellular-resolution, massively parallel artificial control of neuron population activity in the visual system. We examine the system’s ability to drive neuronal activity in optogenetically transduced retinal ganglion cells (RGCs) of pharmacologically or genetically blinded retinas, and demonstrate that it combines single-cell resolved controllability with millisecond-scale precision across a large population of neurons, where the degree of overlap of the projected optical patterns with the cells’ somata defines the probability and temporal precision of RGCs’ firing. Physical performance of the holographic system A schematic diagram of the experimental holographic system is described in Fig. 1a . Polarized laser light from a blue laser is expanded, modulated by a computer-controlled ferroelectric liquid-crystal SLM and imaged onto the back aperture of an inverted microscope objective (TE-2000U, X10 and X4 objectives, Nikon, Japan). The resulting light patterns in the Fourier (sample) plane are used to photo-stimulate retinal nerve cells, and the resulting activity patterns are recorded using a transparent planar microelectrode array. The binary patterns (0 or π phase shift) lead to a mirror-symmetric pattern which is truncated, together with the zero order, by a square slit placed outside the microscope’s camera port. The resulting effective fields of stimulation measure 600 μm or 1.5 mm squared through X10 and X4 objectives, respectively (for λ =473 nm; ~670 μm and ~1680 μm squared, respectively, for λ =532 nm). Within this field, there is independent access to 220 × 230 (partially overlapping) stimulation pixels whose basic point spread function (PSF) has a Gaussian profile ( Fig. 1a ). The spot’s dimensions allow for sub-cellular resolution targeting when targeted cells (ChR2-expressing RGCs) are arranged in a single layer, and can be changed by changing the objective or more finely matched to the cellular dimensions by inversely resizing the laser’s beam diameter (≥4 μm laterally and ≥50 μm axially, Fig. 2a ). As the SLM discretely samples space with square pixels, the diffraction efficiency is spatially varying with a 3D sinc-shaped envelope ( Fig. 2b ). The effective non-uniformity that results in the 2D SF can be compensated by multiplying each point by a weight that is inversely proportional to this spatial sinc function ( Fig. 2c ). In CGH, the total power delivered to the sample is distributed only between the projected points and hundreds to several thousand can be illuminated simultaneously at effective ChR2 stimulation intensity levels with as low as 700 μW of projected power ( Fig. 1b ); the intensity of each point can also be fully modulated by weighting the total intensity between the projected points ( Fig. 1c ). Finally, the temporal resolution of the system is determined by the SLM refresh rate—0.5 ms for this rapid, ferroelectric SLM-based system ( Fig. 1d , rise and fall times of ~50 μs). This ultra-high rate (2,000 holograms per second) can be used for multiplexing large numbers of different holograms, or alternatively for averaging out holographic noise from a single hologram [28] and/or to project multiple different colours for excitation of multiple optogenetic probes [2] , [22] . 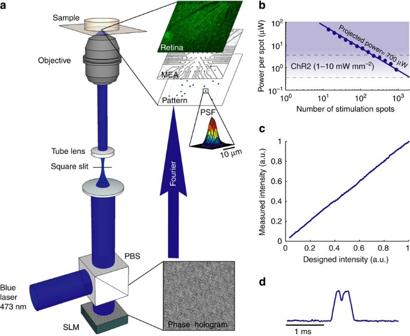Figure 1: Holographic retinal photo-stimulation system. (a) A laser beam is projected through a polarizing beam splitter onto a ferroelectric (binary phase) SLM. The SLM is imaged through a square slit onto the objective lens’ entrance aperture, and Fourier-transformed into a sparse pattern at the focal plane (inset: PSF for a 10 × objective). The light pattern excites ChR2-expressing retinal neurons whose responses are recorded using a multielectrode array. (b) The light flux delivered to the sample plane (~700 μW) is diffractively divided among stimulation spots; power per spot decreases monotonically with increasing spot counts. Even at this low flux, hundreds to thousands of stimulation spots can be generated with the nominal intensity level required for optogenetic stimulation. (c) Analog control of individual spot intensity obtained by appropriately weighing the desired pattern during hologram calculation. (d) Sub-millisecond temporal profile of a single binary frame. Figure 1: Holographic retinal photo-stimulation system. ( a ) A laser beam is projected through a polarizing beam splitter onto a ferroelectric (binary phase) SLM. The SLM is imaged through a square slit onto the objective lens’ entrance aperture, and Fourier-transformed into a sparse pattern at the focal plane (inset: PSF for a 10 × objective). The light pattern excites ChR2-expressing retinal neurons whose responses are recorded using a multielectrode array. ( b ) The light flux delivered to the sample plane (~700 μW) is diffractively divided among stimulation spots; power per spot decreases monotonically with increasing spot counts. Even at this low flux, hundreds to thousands of stimulation spots can be generated with the nominal intensity level required for optogenetic stimulation. ( c ) Analog control of individual spot intensity obtained by appropriately weighing the desired pattern during hologram calculation. ( d ) Sub-millisecond temporal profile of a single binary frame. 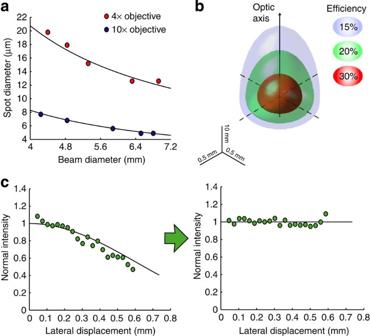Figure 2: Physical performance of the photo-stimulation system. (a) The inverse dependence of the stimulation spot diameter on the beam diameter at the objective back aperture. Red and blue points represent measured spot sizes obtained with X4 and X10 objective lenses, respectively. Solid lines indicate an inverse relation fit. (b) A 3D visualization of the stimulation volumes accessible by the binary-phase holographic system with a X10 objective, for diffraction efficiencies greater than 15% (blue), 20% (green) and 30% (red). (c) The spatially varying diffraction efficiency due to the rectangular SLM pixel shape causes spot intensity to decrease with increasing lateral displacement (green points, left plot), which coincides with theoretical prediction of a sinc-shaped envelope (solid line). Compensation of this effect is achieved by inversely weighing each spot during hologram calculation, resulting in improved uniformity (green points, right plot) close to a constant value (solid line). Full size image Figure 2: Physical performance of the photo-stimulation system. ( a ) The inverse dependence of the stimulation spot diameter on the beam diameter at the objective back aperture. Red and blue points represent measured spot sizes obtained with X4 and X10 objective lenses, respectively. Solid lines indicate an inverse relation fit. ( b ) A 3D visualization of the stimulation volumes accessible by the binary-phase holographic system with a X10 objective, for diffraction efficiencies greater than 15% (blue), 20% (green) and 30% (red). ( c ) The spatially varying diffraction efficiency due to the rectangular SLM pixel shape causes spot intensity to decrease with increasing lateral displacement (green points, left plot), which coincides with theoretical prediction of a sinc-shaped envelope (solid line). Compensation of this effect is achieved by inversely weighing each spot during hologram calculation, resulting in improved uniformity (green points, right plot) close to a constant value (solid line). Full size image Characterization of ChR2-expressing RGCs responsiveness To determine the stimulation conditions required for selectively exciting ChR2-expressing RGCs, we first characterized the responses to long-duration (1 s) uniform wide-field stimuli under varying illumination and pharmacological conditions. Retinas were isolated from transgenic mice that have normal photoreception and also express ChR2 in their RGCs (under a Thy1.2 promoter). Robust natural light-evoked responses to low-intensity illumination pulses were observed ( Fig. 3a–c and Supplementary Fig. S1 ), and were abolished when both on- and off-transduction pathways to the RGCs were pharmacologically blocked (48/51 cells, see exceptions in Fig. 4 ). Robust responses were retrieved when the illumination power was increased by over an order of magnitude, to nominal levels required to selectively excite the ChR2-expressing RGCs (>1 mW mm −2 ). In contrast, light-evoked responses were not seen in control pharmacologically blocked wild-type retinas lacking ChR2 ( Fig. 3b and Supplementary Fig. S1b ), even when illumination intensities were gradually increased to much higher levels (>10 mW mm −2 ). The ChR2-mediated responses were blocked after applying Tetrodotoxin, a selective voltage-gated sodium channel blocker, ruling out direct photoelectric electrode polarization ( Supplementary Fig. S1a ). Next, we characterized the ChR2-mediated responses to varying light intensities ( n =51 cells). The characteristic response curve was sigmoidal on a log-intensity scale, and was fit by a logistic function with 48% response activation at 1 mW mm −2 ( Fig. 3d ). The latency to first spike was a monotonically decreasing function best fit by a power-law dependence on light intensity (exponent: −0.77), reaching down to 23.3 ms for intensities of 2.6 mW mm −2 ( Fig. 3e ). In nearly all cases, the ChR2-mediated responses had characteristic spiking waveforms that were very similar to their corresponding visually evoked waveforms ( Fig. 3f ). 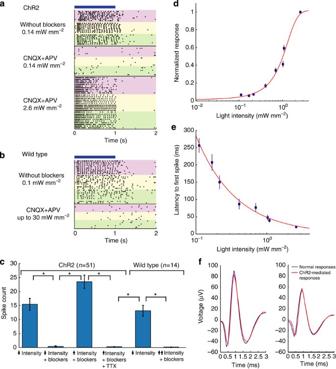Figure 3: Neuronal responses to full-field flashes. (a) Response Raster plots of three units (colour coded) from a ChR2-expressing mouse. The second-long illumination flashes (solid blue line) initially evoke normal visual responses (top) which are blocked by a pharmacological cocktail (middle). Responses (putatively to direct ChR2 excitation) are restored at a higher illumination level (bottom). (b) In wild-type retinas, normal visual responses are evoked, but not seen in pharmacologically blocked retinas even at much higher illumination levels. (c) Summary statistics for neurons from ChR2-expressing (n=51) and wild-type retinas (n=14). Intensities:↓low (0.1–0.15 mW mm−2),↑ high (~2.6 mW mm−2), ↑↑ very high (<30 mW mm−2). Error bars represent s.e.m. values. Significantly different responses are marked by asterisks (two-tailed Student’st-test,P<0.0001). (d,e) Normalized responses and latencies (mean±s.e.m.,n=52 units from single retina) for flashes with varying illumination levels. (f) Comparison of mean extracellular spike waveforms measured in two representative ChR2 units in response to low-intensity (normal vision) and high-intensity (pharmacologically blocked) illumination flashes. Figure 3: Neuronal responses to full-field flashes. ( a ) Response Raster plots of three units (colour coded) from a ChR2-expressing mouse. The second-long illumination flashes (solid blue line) initially evoke normal visual responses (top) which are blocked by a pharmacological cocktail (middle). Responses (putatively to direct ChR2 excitation) are restored at a higher illumination level (bottom). ( b ) In wild-type retinas, normal visual responses are evoked, but not seen in pharmacologically blocked retinas even at much higher illumination levels. ( c ) Summary statistics for neurons from ChR2-expressing ( n =51) and wild-type retinas ( n =14). Intensities: ↓ low (0.1–0.15 mW mm −2 ),↑ high (~2.6 mW mm −2 ), ↑↑ very high (<30 mW mm −2 ). Error bars represent s.e.m. values. Significantly different responses are marked by asterisks (two-tailed Student’s t -test, P <0.0001). ( d , e ) Normalized responses and latencies (mean±s.e.m., n =52 units from single retina) for flashes with varying illumination levels. ( f ) Comparison of mean extracellular spike waveforms measured in two representative ChR2 units in response to low-intensity (normal vision) and high-intensity (pharmacologically blocked) illumination flashes. 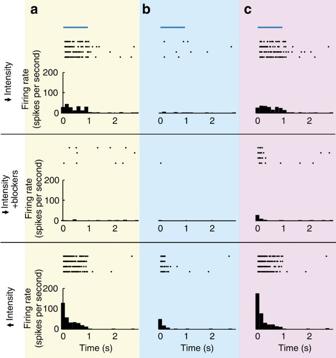Figure 4: Categorization of RGCs responses to wide-field stimuli. Of 93 channels (n=2 ChR2-expressing retinas) which responded to high-intensity blue light (after application of blockers). (a) In 66 units, the response was abolished with application of blockers and intense response was restored with high-intensity light stimulation (as inFig. 2a). (b) A total of 15 units did not respond to lower light stimuli (0.08–0.17 mW mm−2) with and without blockers, but responded to intense blue light. (c) In 12 units, a shorter and weaker response was still observed after application of blockers and a more robust response was later observed to high-intensity light. These responses may indicate a higher concentration of ChR2 channels, or a higher underlying excitability of these cells.↓-low (0.1–0.15 mW mm−2),↑-high intensities (~2.6 mW mm−2). Full size image Figure 4: Categorization of RGCs responses to wide-field stimuli. Of 93 channels ( n =2 ChR2-expressing retinas) which responded to high-intensity blue light (after application of blockers). ( a ) In 66 units, the response was abolished with application of blockers and intense response was restored with high-intensity light stimulation (as in Fig. 2a ). ( b ) A total of 15 units did not respond to lower light stimuli (0.08–0.17 mW mm −2 ) with and without blockers, but responded to intense blue light. ( c ) In 12 units, a shorter and weaker response was still observed after application of blockers and a more robust response was later observed to high-intensity light. These responses may indicate a higher concentration of ChR2 channels, or a higher underlying excitability of these cells. ↓ -low (0.1–0.15 mW mm −2 ), ↑ -high intensities (~2.6 mW mm −2 ). Full size image Patterned optogenetic stimulation of intact retinas To study the spatio-temporal characteristics of the optogenetic responses, we directly stimulated ChR2-expressing RGCs with sparse pseudo-random, uniformly distributed, point patterns generated by the holographic system ( Fig. 1a ). These experiments included the pharmacologically blinded retinas described above ( n =7) as well as retinas isolated from natively blind ChR2-expressing transgenic mice (n=4) which resulted from crossing together mouse lines with retinal degeneration and with ChR2-expressing phenotypes [29] ( Fig. 5 ). Patterns projected through a X10 objective lens had focal point spreads ( Fig. 1a ) that covered enough of the cellular surface to drive responses in a large subset of the ChR2-responsive units (19/51 in the experiment shown in Fig. 5a . ), but were much smaller than RGCs dimensions, so as to allow spatially selective responses to be finely mapped (~5.5 μm full-width at half-maximum versus ~20 μm cell diameter). The resulting ‘stimulation fields’ (SFs—termed in analogy to receptive fields, n =219 in the 11 retinas) typically matched the size and the shape of RGC somata and in the large majority of cases exactly overlapped with the somata of fluorescently identified RGCs ( Fig. 5b ). Interestingly, in a significant minority (~20%) of the SFs, we somewhat paradoxically did not observe an underlying soma ( Fig. 5c , n =45/219), although the size and shape were of the same dimensions. This could suggest that lower levels of ChR2-eYFP expression are sufficient for efficient excitation than for fluorescent detection, and that perhaps more RGCs are light excitable than previously reported [29] . In a few other cases (13/219, not shown), we observed large, diffuse fields that in general overlapped with an observed cluster of cells. Overall, the mean SF had a cellular-scale diameter of ~20 μm ( Fig. 5d , average of n =202 unimodal SFs). 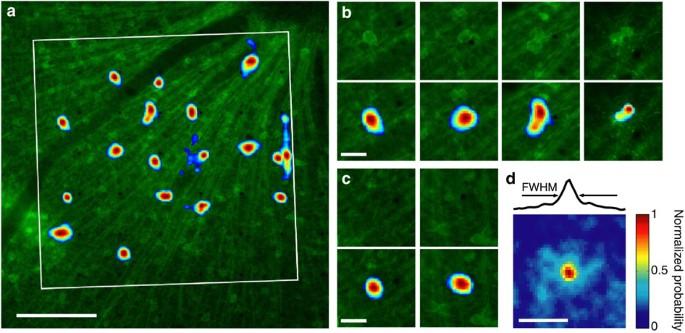Figure 5: Cellular-resolution optogenetic ‘retinal stimulation fields’. (a) Fluorescent image of retina and multielectrode array (black dots) with superposed distribution of SFs (estimated using spike-triggered averaging of pseudo-random holographic patterns with 20 spots each). Scale bar, 200 μm (b,c) Examples where retinal SFs match (b) or do not correspond to (c) visualized ChR2-eYFP-expressing RGCs. Scale bars, 20 μm (d) Mean SF spatial distribution (n=202 units from 11 retinas). Scale bar, 50 μm. Figure 5: Cellular-resolution optogenetic ‘retinal stimulation fields’. ( a ) Fluorescent image of retina and multielectrode array (black dots) with superposed distribution of SFs (estimated using spike-triggered averaging of pseudo-random holographic patterns with 20 spots each). Scale bar, 200 μm ( b , c ) Examples where retinal SFs match ( b ) or do not correspond to ( c ) visualized ChR2-eYFP-expressing RGCs. Scale bars, 20 μm ( d ) Mean SF spatial distribution ( n =202 units from 11 retinas). Scale bar, 50 μm. Full size image Next, we explored the response characteristics to holographic excitation patterns that closely match neuronal dimensions. We measured responses of ChR2-transduced neurons from blind mice to projected pseudo-random arrangement of spot patches ( Fig. 6a ). The patches used in these experiments were arranged in disk-like geometries with diameters of 3, 5, 7 and 9 pixels. As is generally the case in the holographic projection of contiguous shapes, the projected circular patches suffered from severe distortion, as a result of holographic speckle, which we eliminated by shift-averaging [28] , that is, by sequentially projecting 24 periodic 2D cyclic shifts of this hologram each for 0.5 ms ( Fig. 6a ). By projecting spot patches in a large number of locations, we were able to characterize the effect of varying the cellular coverage by the projected patch ( Fig. 6b ). Qualitatively, increasing either coverage or light intensity resulted in stronger responses with shorter response latencies in single cells ( Fig. 6c ). Across the population of recorded units, the dependence of mean response latency ( Fig. 6e ) and mean firing probability ( Fig. 6f ) on cellular coverage were respectively fit by an inverse power law: ( R 2 =0.91–0.96) and by: ( R 2 =0.97–0.99). At the highest level of cellular coverage (90–100%), the median firing probabilities (which were generally larger than the means), were as high as 89.3% (10–30 mW mm −2 ), 85.2% (7–10 mW mm −2 ) and 71% (2–7 mW mm −2 ), respectively, while median latencies were 11, 14.5 and 18.4 ms, respectively. Moreover, in preliminary experiments, we observed that patch-based stimulation allows to emulate RGCs visual cellular activity patterns. Isolated retinas from sighted mice were first projected with low-intensity movies (~0.011 mW mm −2 , moving cat), and the resulting visually evoked RGCs’ activity was optogenetically emulated ( Fig. 6g , 1 mW mm −2 ) following pharmacological block and stimulation-field mapping. The resulting emulated activity was significantly correlated with the visual activity pattern target ( R =0.8 in Fig. 6g , note the relatively high spontaneous firing rates in the pharmacologically blocked retinas). 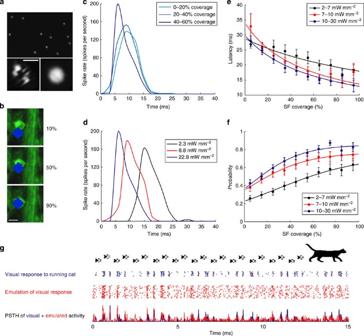Figure 6: Optogenetic photo-stimulation with holographic spot patches. (a) A pseudo-random projection image of spot patches (disk-like arrangement, 5 pixel diameter). Inset: zoomed image of a patch with speckle (left) and a patch after speckle was shift-averaged (right, 24 shifted copies of hologram projected sequentially). (b) Illustration of variable coverage of a cell’s soma by moving a patch around. (c,d) Peri-stimulus time histograms (PSTHs) showing effect of coverage (at 22.8 mW mm−2) and of illumination intensity (at 40–60% coverage) on the responses of a representative unit. (e,f) Spike latency and firing probability as a function of cell coverage (mean±s.e.m.,n=31 units from two retinas). Latency plot is fit with inverse power fit (exponent, −0.77) and probability plot with an exponential saturation line. Time is relative to beginning of stimulation frame. (g) Optogenetic emulation of visual responses. Raster graphs of visually evoked neural activity in response to running cat (blue) and optogenetically emulated neural activity (red). PSTH graphs were calculated and overlaid to illustrate the resemblance between the two point processes. Scale bars, 10 μm. Figure 6: Optogenetic photo-stimulation with holographic spot patches. ( a ) A pseudo-random projection image of spot patches (disk-like arrangement, 5 pixel diameter). Inset: zoomed image of a patch with speckle (left) and a patch after speckle was shift-averaged (right, 24 shifted copies of hologram projected sequentially). ( b ) Illustration of variable coverage of a cell’s soma by moving a patch around. ( c , d ) Peri-stimulus time histograms (PSTHs) showing effect of coverage (at 22.8 mW mm −2 ) and of illumination intensity (at 40–60% coverage) on the responses of a representative unit. ( e , f ) Spike latency and firing probability as a function of cell coverage (mean±s.e.m., n =31 units from two retinas). Latency plot is fit with inverse power fit (exponent, −0.77) and probability plot with an exponential saturation line. Time is relative to beginning of stimulation frame. ( g ) Optogenetic emulation of visual responses. Raster graphs of visually evoked neural activity in response to running cat (blue) and optogenetically emulated neural activity (red). PSTH graphs were calculated and overlaid to illustrate the resemblance between the two point processes. Scale bars, 10 μm. Full size image In summary, we have shown that holographic photo-stimulation could be applied in patterned vision restoration systems where it offers an unprecedented level of control over multi-cellular activity patterns. This diffractive method is uniquely suited for optogenetic excitation by allowing parallel stimulation of multiple points at high local light intensities with millisecond-scale temporal precision, and can also be combined with sophisticated optogenetic strategies requiring multi-colour excitation [8] . As the generation of each spike requires threshold light energies of only a few nanojoules, complex spatio-temporal neuronal activity patterns containing thousands to millions of actions potentials per second can potentially be elicited using projected laser powers as low as a few milliwatts. Our results provide new quantitative relationships between control parameters (cellular coverage and intensity) and effectiveness measures of cellular excitation, which generalize across experimental conditions (wide field versus patterned). They indicate that effective excitation of ChR2-expressing RGCs (with probability as high as 90% and latencies of ~11 ms) occurs when their soma is illuminated with a short, patch of light, which exactly matches somatic location and dimensions (>70% coverage being nearly as effective). Projection of such contiguous patches of light using CGH techniques presents a unique challenge because of the appearance of ‘holographic speckle’. The projected patterns were effectively de-speckled here using ‘shift-averaging’ [28] , [30] —sequential projection of cyclically shifted versions of the same hologram. Because shift-averaging removes speckle deterministically [28] , and the display’s projection rate is 2,000 frames per second, effective patch de-speckling requires only a few milliseconds (2–12 ms in these experiments), allowing for very high effective temporal resolution, which would practically probably be limited by other factors (for example, video processing, hologram computation and optogenetic probe response times). Holographic speckle has emerged as an important issue in the implementation of diffractive photo-stimulation systems [31] , and it is important to note several alternative designs for circumventing this issue including the use of Generalized Phase Contrast [26] , hybrid holographic-mechanical projection systems (that is, rotating diffusers [32] or mechanically vibrated smearing of point patterns [33] ). Other possibilities for speckle reduction are the use of temporally and/or spatially incoherent light sources. Incoherent light sources such as LEDs can be combined with SLMs to generate desired light patterns using optical transfer function design [34] and CGH [35] . The cellular level of precision demonstrated—the mean SF diameter ( Fig. 5d ) was ~20 μm (corresponding to ~0.7° and ~0.07° of visual angle in mice and humans, respectively), contrasts with a previous report, which argued that ChR2 cellular excitation requires very large (>100 μm) excitation spots [12] , [14] . A recent report suggested that a retinal prosthetic system with cellular activity emulating natural RGCs encoding strategies, could underlie the restoration of vision to normal performance levels [9] . However, that report did not attempt to characterize their display's effective spatial and temporal resolution and effectiveness in controlling neuronal activity at the fine scale of single cells and spikes. The use of mini-DLP (Digital Light Processor, micromirror-based) displays in the generation of sparse spatial-temporal RGCs activity patterns [15] is inherently power inefficient, as most of the light source's light is blocked—a potentially important issue for practical implementation. Our results thus suggest that holographic photo-stimulation systems could potentially be used in efficient high-acuity in vivo vision interfaces with single-cell resolution. To address this possibility, we have recently begun exploring cellular-resolved in vivo retinal imaging [36] and its integration with holographic projection systems for cellular-resolution optogenetic targeting ( Fig. 7 ). Although here we did not utilize the inherent 3D projection capability of holographic photo-stimulation, it may have a major role in the applicability of this technology, as unlike in rodents, human RGCs are arranged in a 3D, multi-layered (2–5 layers) structure around the foveal pit, where high-acuity vision restoration may be most crucial [37] (the expected visual acuity in human vision restoration is a complex function of the para-foveal and peri-foveal 3D distribution of optogenetically transduced surviving RGCs, their receptive field structures and the optical system’s resolution performance). The projected phase waveform from the SLM can also potentially be used for cancelling corneal aberrations [38] . However, the practical engineering of a high-acuity prosthetic system is highly non-trivial and will require the integration of real-time image-processing for emulating the ganglion-cell encoding of the visual stimuli [39] , [15] (which generally includes a diversity of response types [40] ), high-resolution eye-tracking [39] and real-time hologram computations. Major challenges also remain on the optogenetic probe engineering front—including testing of strategies for safe and effective cellular transfections [7] , and the exploration of favourable red-shifted alternatives to ChR2 (whose excitation peak is effectively absorbed by pigments of the macula lutea in humans [41] ). 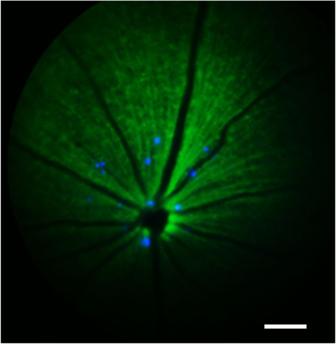Figure 7:Holographic stimulation pattern projection onto a ChR2-eYFP-expressing retinain vivo. Fundus fluorescence image of ChR2-eYFP expressing mouse retinal neurons (green) superimposed with fluorescence image of holographic illumination pattern on the retina (blue). Pattern spot sizes were less than 40 μm. Scale bar, 250 μm. Figure 7: Holographic stimulation pattern projection onto a ChR2-eYFP-expressing retina in vivo . Fundus fluorescence image of ChR2-eYFP expressing mouse retinal neurons (green) superimposed with fluorescence image of holographic illumination pattern on the retina (blue). Pattern spot sizes were less than 40 μm. Scale bar, 250 μm. Full size image Our results also suggest that the combination of optogenetic holography and multielectrode array recording technology already offer some exciting, yet-unexplored applications, such as providing ‘ground-truth’ reference measurements for resolving ambiguities in neuronal spike sorting ( Fig. 3f ). By allowing this level of spatial-temporal control over neuronal dynamics, holographic-patterned photo-stimulation could allow the realization of optical ‘network clamps’, with possible wide-ranging applications for shedding new light on fundamental problems in neuroscience research as well as in medical applications. The holographic system The design and characteristics of holographic stimulation systems, including the one used here were previously described and analysed in-depth in Golan et al . [22] Our optical set-up is based on a blue diode-pumped solid state (DPSS) laser (473 nm; VA-I-N-473, 50 mW, Viasho, China). Beam expansion is performed by a 1:4 Galilean telescope. The diameter of the expanded beam is ~9.5 mm at full-width at half-maximum. The expanded beam is reflected by a polarizing beam splitter onto the SLM. The SLM is a ferroelectric liquid-crystal micro-display (SXGA-R3, ForthDD, Scotland) with a 33° switching angle and a 13.6-μm pixel pitch. The incoming polarized light incident on each pixel is rotated with either a positive or negative switching angle, dependent on the pixel state. The polarizing beam splitter transfers only the perpendicular component of the outcoming light, effectively creating a phase-only binary hologram with [0,π] modulation. Only the central 512 × 512 pixels of the SLM are used for displaying the hologram, to speed up calculations, at the expense of a larger spot size. The modulated wavefront is imaged by a Keplerian 2:1 telescope to the back aperture of a microscope objective, to avoid vignetting. The telescope de-magnification increases the maximal diffraction angle. The objective is a part of an inverted microscope (TE-2000U, Nikon, Japan), and the second lens of the telescope is the microscope tube-lens. The first lens of the telescope creates an intermediate image outside the microscope, where unwanted diffraction orders are blocked by the placement of a rectangular aperture stop ( Fig. 1a ). Different microscope objectives may be used to obtain different combinations of resolution, field and spot size. In this work, we used a CFI Achromat DL X10 (NA=0.25, 20 mm focal length, Nikon, Japan) to obtain a 0.6 × 0.7 mm field. A CCD camera (Hamamatsu C8484-05G, Japan) was attached to the microscope, and used to record the resulting stimulation patterns, as well as fluorescence and bright-field images of the neural specimens. This was also used to align the stimulation pattern with the specimen. Experimental animals and retina preparation The animal experiments and procedures were approved by the Institutional Animal Care Committee at Technion—Israel Institute of Technology and were in accord with the National Institutes of Health Guide for the Care and Use of Laboratory Animals. Adult mice from two transgenic lines were used: sighted mice expressing ChR2-eYFP under a Thy1.2 promoter (4 weeks–4 months old, strain: B6.Cg-Tg(Thy1-COP4/EYFP)18Gfng/J, The Jackson Laboratory, USA), and cross-bred rd1/ChR2-eYFP mice (2–4 months old) that progressively develop outer retinal degeneration. Details on the cross-bred line’s derivation, functional and structural characterizations and of the retinal isolation procedure appear in the Supplementary Methods . Wide-field stimulation Wide-field stimulation was achieved with a blue DPSS laser (473 nm, 50 mW, Viasho Lasers, China) that was coupled to an optical fibre with a 200-μm core diameter (BFL37-200-custom, Thorlabs). The light was homogenized with a circular light shaping diffuser with a 15° angle (10Dkit-C1, Newport), and was projected from below the sample, close to the RGCs. The intensity of the stimulating flash was controlled using neutral density filters (FRQ-ND, Newport). The duration of the wide-field flashes was controlled by an electro-mechanical beam shutter (SH05+SC10 shutter controller, Thorlabs) which was placed at the laser's output. Basic stimulation protocol for initial establishment of RGCs’ responses was 1 s of light ON and 9 s of light OFF. Holographic-patterned stimulation Binary holograms were calculated by the ‘Randomal Superposition’ method (SR) [42] (which works well for non-symmetric patterns [22] ). The target stimulation pattern was multiplied by a random phase mask, then inverse Fourier transformed. The binary phase was obtained from the inverse transform by the following binarization transformation: Where x i , y j are the pixel centre coordinates. The holograms were calculated by an Intel Core2 Q9300 2.5 GHz personal computer. Numerical processing was done by a MATLAB software (Mathworks, USA). The hologram sequence was transferred to the SLM through a DVI interface. Precise control over video timing was achieved by using the Psychtoolbox extension [43] . For SF characterization, pseudo-random, uniformly distributed holograms containing 20 points each, were projected under optimal intensity conditions (which were previously determined during wide-field stimulation), with 1 or 3 frames ON duration and 11 frames OFF duration (~11.8 ms each frame). In most cases, 10 min of movie projection were enough to establish the SF size and shape; however for smoother results, we projected the patterns for 30 min. In another subset of experiments, the spots were expanded into semi-circular patches of 3, 5, 7 and 9 pixels in diameter ( Fig. 6b ). To eliminate the speckle phenomena, a shift averaging algorithm was applied [28] and we sequentially projected 24 2D cyclic shifts of each hologram (0.5 ms for each shift resulting with total of ~12 ms for a single averaged frame) ( Fig. 6a ). RGCs were mapped using random patterns with higher intensity (~0.58 mW mm −2 ). Preliminary experiments for optogenetic emulation of visual activity ( Fig. 6d ), used retinas from the sighted ChR2-expressing mice ( n =4), and consisted of four steps. First, visual responses to a short movie of a running cat projected through the SLM with low intensity (~0.011 mW mm −2 ) were recorded. Next, we applied synaptic pharmacological blockers to the RGCs and used intense patterns (1 mW mm −2 ) for optogenetic SFs mapping. Third, emulation pattern holograms were calculated based on the recorded temporal activity of the corresponding cells during the first 15 s of the movie (step 1)—the mapped SFs were excited using circular patches of 9 pixels (~16 μm diameter) with 2 ms duration per action potential (2 × 2 shift-averaged holograms lasting 0.5 ms each). Finally, the calculated holograms (7,500 per movie, 40 repeats) were projected onto a blinded retina and electrophysiological activity was recorded. Electrophysiology and data analysis Evoked retinal activity was recorded using a transparent MEA with 60 electrodes of 10 μm in diameter and 100 μm spacing (100/10-ITO, Multi Channel Systems MCS Gmbh). To form a recording chamber (in which the tissue was placed), a polycarbonate cylinder was glued onto the MEA using a transparent RTV-1 silicone rubber (Wacker, Elastosil E41). The RGCs were kept in close proximity to the electrodes using a specially developed holder and continuously perfused with oxygenated Ringer’s solution at room temperature. The recording was made in the presence of CNQX (25 μM) and APV (25 μM) to eliminate photoreceptor mediated responses of RGCs. The experiments lasted about 6 h and RGCs remained stably active during this time period. The presence of photoelectric artifacts was ruled out by applying Tetrodotoxin, 1 μM (no. 1069, Tocris Bioscience) at the end of each experiment. The signals were sampled at 10 KHz using a data acquisition board (E6071, National Instruments) and were recorded, displayed and analysed (off-line) using custom software developed in MATLAB (Mathworks, USA). Spike sorting (using WaveClus [44] ) was performed in only a subset of experiments, as it had little effect on the results. The significance of spike count difference under wide-field stimulation conditions was determined using a two-tailed Student’s t -test ( P <0.0001). SFs were mapped by spike-triggered averaging of the projected frames that were first convolved with the PSF of the holographic spot. Averaged frames were normalized and filtered with a subtle 2D symmetrical Gaussian filter ( σ =1, diameter of 7 pixels). SF maps were generated using an automatic segmentation algorithm after averaged background values were subtracted and a threshold was applied to remove the remaining irrelevant background values. The SF maps were aligned with the retinal fluorescence images using a calibration grid holographic image taken at the beginning of each experiment. In few experiments, minor rescaling was required to properly align the maps due to a natural relaxation of the retinal tissue during a prolonged experiment that resulted in a shift of the RGCs on the MEA. The mean SF was extracted by averaging all the SFs aligned to their centre of mass. The in-vivo holographic system We constructed a custom system based on the design of the in-vitro holographic system described above, combined with an endoscope-based small animal fundus imager [36] , [45] . To acquire fundus fluorescence images, we used a white light illumination source (Intensilight C-HGFI, Nikon, Japan), a blue excitation filter (XF1068, Omega Optical), a green emission filter (MF535-22, Thorlabs), and an SLR camera (D5000 with Nikkor 80–200 F/2.8 AF-D lens, Nikon, Japan). The imaging resolution (~20 μm) was derived as described in Schejter et al . [36] The holographic pattern was generated using a ferroelectric liquid-crystal micro-display (SXGA-R3, ForthDD, Scotland) and a blue DPSS laser light source (473 nm; Lambdapro Technologies, China), and projected through the back aperture of the endoscope using a 3:1 demagnifying Kepler telescope. The dimensions of spots projected on the optic disc were measured (a relatively large area of uniform expression—spot size was compensated for the imaging PSF). How to cite this article: Reutsky-Gefen, I. et al . Holographic optogenetic stimulation of patterned neuronal activity for vision restoration. Nat. Commun. 4:1509 doi: 10.1038/ncomms2500 (2013).